Single-molecule analysis of transcription factor binding at transcription sites in live cells Although numerous live-cell measurements have shown that transcription factors (TFs) bind chromatin transiently, no measurements of transient binding have been reported at the endogenous response elements (REs) where transcription is normally induced. Here we show that at endogenous REs the transcriptionally productive specific binding of two TFs, p53 and the glucocorticoid receptor (GR), is transient. We also find that the transient residence times of GR at endogenous REs are roughly comparable to those at an artificial, multi-copy array of gene regulatory sites, supporting the use of multi-copy arrays for live-cell analysis of transcription. Finally, we find that at any moment only a small fraction of TF molecules are engaged in transcriptionally productive binding at endogenous REs. The small fraction of bound factors provides one explanation for gene bursting and it also indicates that REs may often be unoccupied, resulting in partial responses to transcriptional signals. Many different live-cell imaging experiments have found that site-specific transcription factors (TFs) typically interact transiently with chromatin [1] , [2] . Such transient binding has been detected by multiple fluorescence light microscopy approaches, including fluorescence recovery after photobleaching (FRAP), fluorescence correlation spectroscopy (FCS) and single-molecule tracking (SMT). However, despite more than a decade of work it remains uncertain how TFs bind in vivo at their endogenous response elements (REs), where transcriptional regulation normally occurs. This uncertainty arises for three reasons. First, the vast majority of live-cell measurements of in vivo TF binding have been made at random locations in the nucleus [1] , [2] . Unfortunately, in these experiments it is not known what fraction of the bound TF molecules are at endogenous REs, since there is a vast excess of non-specific sites at which the TF might also bind. As a result, it is likely that much of this transient binding reflects non-specific interactions with chromatin, which are expected to be transient (reviewed in ref. 2 ). The second reason that transient binding at endogenous REs remains a point of contention is that the only definitive measurements of such specific-site binding have come from experiments performed at tandem gene arrays [3] , [4] , [5] , [6] , where specific sites are clustered in repeats numbering from 10 to 1,000 fold. In these cases, a substantial fraction of specific-site binding will contribute to the live-cell binding measurement. However, the array systems are at best unusual situations and at worst artificial constructs, and so they may not accurately reflect typical endogenous REs. The third reason for the uncertainty about transient binding at endogenous REs is that to date the only measurement of TF residence times at such sites has shown the opposite, namely very stable binding. The yeast TF Rap1 exhibits chromatin residence times ranging from 30 to 90 min at hundreds of different single-copy genes, as determined using a chromatin-immunoprecipitation (ChIP) assay that measures the rate at which an induced form of Rap1 marked with one epitope displaces an endogenous form of Rap 1 marked with a second epitope [7] . In addition to the uncertainty about whether some TFs bind transiently at endogenous REs, none of the preceding approaches have been able to address the question of what fraction of the TF molecules in a nucleus are engaged in transcriptionally productive interactions at endogenous REs. This information is required to determine if the complete set of gene targets for a given TF are fully occupied within each cell nucleus. To address these limitations, we have used a GFP-tagged polymerase II to define transcriptionally productive domains in the nucleus [8] , [9] . We performed SMT within and outside of these domains to determine the residence times of two TFs, p53 and the glucocorticoid receptor (GR) [10] , [11] , at their endogenous REs. With this approach, we identify a subfraction of TFs unique to transcriptionally productive domains that exhibits markedly longer dwell times compared to the same TFs outside of those domains. We conclude that this unique subfraction reflects binding at transcriptionally productive endogenous REs. We find that the mean residence times of this unique sub-fraction are 3.5 s for p53 and 8.1 s for GR, suggesting that transcriptionally productive interactions are relatively transient at endogenous REs. We also find that the size of this unique subfraction is small (only a few percent of total p53 or GR molecules), indicating that at any moment only a sparse number of TF molecules are involved in transcriptionally productive interactions, a result that has important implications for both transcriptional bursting and regulation of cellular gene networks. Visualizing single-molecule TFs We detected single TF molecules in live cell nuclei by transient transfection of p53 or GR fused to the HaloTag [12] , [13] . Controls showed that the binding dynamics of TFs fused with the HaloTag was comparable to the binding dynamics of TFs fused with the commonly used GFP tag ( Supplementary Fig. 1a–d ). We kept the expression levels of transfected TFs very low to limit the total number of fluorescently tagged molecules. Westerns of GR transfected cells showed that the HaloTag-GR was significantly underexpressed relative to the endogenous GR in the 3134 mouse adenocarcinoma cells used for SMT of GR ( Supplementary Fig. 2 ). Comparable transfection conditions were used for the p53 SMT experiments, which were performed in the p53-null human cell line H1299. Note that we examined p53 binding in the absence of stress or DNA damage, as previous studies have shown that p53 can still bind and induce transcription of genes under these conditions [14] , [15] , [16] . To confirm this under our experimental conditions, we used PCR with reverse transcription in unstressed cells to demonstrate mRNA induction with the HaloTag version of p53 ( Supplementary Fig. 3 ). To fluorescently tag the TFs, we incubated transfected cells with the membrane-permeable HaloTag tetramethylrhodamine (TMR) ligand and then washed extensively to remove unbound ligand. We observed the TMR-tagged molecules of p53 or GR with a microscope equipped with highly inclined laminated optical sheet illumination (HILO) [17] . We could visualize single molecules of p53 or GR as bright diffraction-limited spots within live nuclei ( Fig. 1 ). To identify chromatin-bound molecules, we collected time-lapse images spaced by 0.2 s (see the example in Supplementary Movie 1 ), which enables monitoring of longer binding events without introducing excessive observational photobleaching. In our time-lapse movies, stably bound molecules remained relatively immobile for multiple frames ( Fig. 1 , yellow arrow), whereas free molecules did not ( Fig. 1 , red trajectory). Some molecules were visible in only one frame and these reflected either completely free molecules or bound molecules with residence times <0.2 s, which in either case could lead to large displacements of the molecule outside of the field of view at the next time point ( Fig. 1 , green arrow). 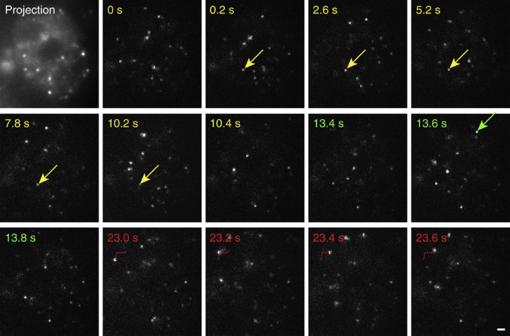Figure 1: Images of GR single molecules in the nucleus of a live cell. HaloTMR-tagged GR molecules at selected time points (upper left corner) are presented from a 60-s movie. Projection of 85 successive timepoints from the movie defines the boundary of the nucleus (first frame). Colour coding in subsequent panels indicates three separate segments of the movie illustrating a bound molecule (yellow—residence time of 10 s), a molecule that appears for only one timepoint (green) and a free molecule that diffuses in the plane of focus (red). Arrows indicate the molecule of interest. The red dotted line indicates the path of the diffusing molecule. Scale bar 1 μm. Figure 1: Images of GR single molecules in the nucleus of a live cell. HaloTMR-tagged GR molecules at selected time points (upper left corner) are presented from a 60-s movie. Projection of 85 successive timepoints from the movie defines the boundary of the nucleus (first frame). Colour coding in subsequent panels indicates three separate segments of the movie illustrating a bound molecule (yellow—residence time of 10 s), a molecule that appears for only one timepoint (green) and a free molecule that diffuses in the plane of focus (red). Arrows indicate the molecule of interest. The red dotted line indicates the path of the diffusing molecule. Scale bar 1 μm. Full size image Tracking TFs within and outside of transcription domains To detect TF binding events within and outside of transcriptionally productive domains, we used single-molecule colocalization microscopy to visualize a previously characterized GFP-tagged component of the polymerase complex (RPB1 (ref. 18) [18] ). We expressed the GFP polymerase at high levels such that we could detect its distribution throughout the nucleus. After fixation and imaging by conventional fluorescence microscopy with camera exposure times of ~1 s, we could detect characteristic polymerase foci that showed a high degree of colocalization with sites of 5-bromouridine 5′-triphosphate (BrUTP) incorporation, demonstrating that these foci marked sites of active transcription ( Fig. 2a–c ). To track red-labelled TFs relative to this polymerase distribution, we imaged live cells with the single-molecule HILO microscope and alternated collection of red and green images, each for a 10-ms exposure with 0.1-s time intervals between the alternate colours. We averaged the GFP-polymerase II time-lapse images to generate a single image that again revealed polymerase foci ( Fig. 2d,e ). These foci identify nuclear domains that should be transcriptionally productive, and conversely also identify regions largely devoid of the polymerase that should be transcriptionally inactive. We tracked single molecules of p53 and GR in the presence of dexamethasone within both types of regions ( Fig. 2f,g and Supplementary Movies 2,3 ), as defined in each case by a 0.6-μm-diameter circle ( Fig. 2e , dotted circles), which was the maximal diameter of the polymerase foci obtained from our time-averaged projection image. 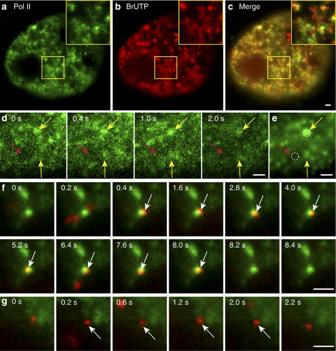Figure 2: Single-molecule tracking within and outside of transcription domains. Fixed cells showing GFP-tagged polymerase II puncta (a) with BrUTP incorporation marking sites of transcription (b). Many polymerase II puncta are sites of BrUTP incorporation (overlay,c). Four time points (shown in the upper left corner) of a GFP-polymerase II movie taken in live cells (d), and the projection image from that movie (e). Yellow arrows indicate examples of polymerase II foci that appear in multiple frames and give rise to well-defined domains in the averaged movie. Red arrow indicates a region largely devoid of polymerase. Dotted circles (0.6 μm diameter) provide examples of regions where single-molecule tracking would be performed. (f) Selected time points from a movie showing association of a single GR molecule (red) with an averaged projection of a polymerase II movie (green). White arrows indicate the frames (0.4–8.0 s) during which the GR molecule remains bound within the transcription domain. (g) Selected time points from a movie showing a bound GR molecule away from a transcription domain, with binding occurring from 0.2 to 2.0 s. Scale bar 1 μm. Figure 2: Single-molecule tracking within and outside of transcription domains. Fixed cells showing GFP-tagged polymerase II puncta ( a ) with BrUTP incorporation marking sites of transcription ( b ). Many polymerase II puncta are sites of BrUTP incorporation (overlay, c ). Four time points (shown in the upper left corner) of a GFP-polymerase II movie taken in live cells ( d ), and the projection image from that movie ( e ). Yellow arrows indicate examples of polymerase II foci that appear in multiple frames and give rise to well-defined domains in the averaged movie. Red arrow indicates a region largely devoid of polymerase. Dotted circles (0.6 μm diameter) provide examples of regions where single-molecule tracking would be performed. ( f ) Selected time points from a movie showing association of a single GR molecule (red) with an averaged projection of a polymerase II movie (green). White arrows indicate the frames (0.4–8.0 s) during which the GR molecule remains bound within the transcription domain. ( g ) Selected time points from a movie showing a bound GR molecule away from a transcription domain, with binding occurring from 0.2 to 2.0 s. Scale bar 1 μm. Full size image We used the tracks from the two different regions to calculate dwell times, namely the time period for which a molecule remains nearly stationary, allowing only for the small movements characteristic of a molecule bound to chromatin (see Methods). We found that the distribution of dwell times outside of transcription domains was similar for both p53 and GR with virtually no dwell times longer than 3–4 s (blue curves in Fig. 3a,b ). In contrast, the distribution of dwell times within transcription domains exhibited an extended tail of longer times that fell to zero by ~15 s for p53 and by ~25 s for GR (red curves in Fig. 3a,b ), suggesting the presence of a unique component with longer dwell times within transcription domains. To determine if these dwell time measurements were radically altered by photobleaching, we also measured dwell times from SMT data for the histone H2B. These dwell time distributions showed a markedly slower fall-off with time ( Supplementary Fig. 4 ), indicating that it is possible to measure much longer dwell times by SMT than those we have measured for p53 and GR. 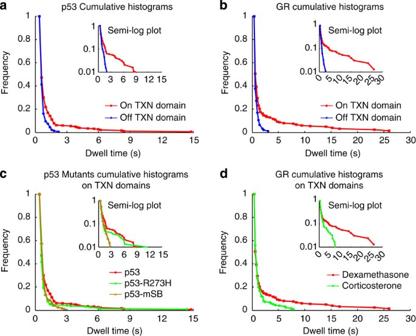Figure 3: Cumulative histograms with semi-log plots (insets). Dwell times of molecules in transcription domains are significantly longer than dwell times of molecules away from transcription domains for both p53 (a) and GR (b). The tail of the histogram for the seven-amino-acid specific-site binding mutant p53 mSB disappears, while a reduction in the height of the tail is seen for the single-amino-acid mutant p53 R273H (c). The tail of the histogram of GR activated with corticosterone fell to zero earlier compared to dexamethasone activation (d). We collected 20–30 time-lapse movies for each experimental condition. From this set of movies we selected 2–3 representative movies in which the number and brightness of the single molecules were optimal for tracking, and from these movies we tracked a total of 400–700 single molecules for each condition. SeeSupplementary Fig. 6for histograms of p53 mSB, p53 R273H and GR outside of transcription domains, andSupplementary Fig. S5for representative fits to these data. Figure 3: Cumulative histograms with semi-log plots (insets). Dwell times of molecules in transcription domains are significantly longer than dwell times of molecules away from transcription domains for both p53 ( a ) and GR ( b ). The tail of the histogram for the seven-amino-acid specific-site binding mutant p53 mSB disappears, while a reduction in the height of the tail is seen for the single-amino-acid mutant p53 R273H ( c ). The tail of the histogram of GR activated with corticosterone fell to zero earlier compared to dexamethasone activation ( d ). We collected 20–30 time-lapse movies for each experimental condition. From this set of movies we selected 2–3 representative movies in which the number and brightness of the single molecules were optimal for tracking, and from these movies we tracked a total of 400–700 single molecules for each condition. See Supplementary Fig. 6 for histograms of p53 mSB, p53 R273H and GR outside of transcription domains, and Supplementary Fig. S5 for representative fits to these data. Full size image Specific binding of TFs within transcription domains To test if dwell times within transcription domains contained a unique component, we fit the data with one- or two-component exponentials, which are predicted theoretically to describe distributions of binding residence times [13] . Although we varied the fitting conditions, we always obtained consistent results ( Supplementary Tables 1,2 and Supplementary Fig. 5 ). A single-component model explained the p53 and GR data outside of transcription domains with a mean dwell time of ~0.3 s, while a two-component model was required to fit the data within transcription domains, with the fast component yielding a comparable mean dwell time of ~0.3 s and the slow component yielding a dwell time of 3.5±1.6 s for p53 and 8.1±2.1 s for GR. The shorter mean dwell time of ~0.3 s reflects a mix of slowly diffusing molecules and very transiently bound molecules. However, the longer dwell times that were unique to transcription domains reflect chromatin residence times since the odds of a free molecule remaining in place for >1 s is very small (<1 in 10 −7 for a 1-MDa TF complex). These long residence times within transcription domains occurred for only a small fraction, namely 5.5±1.5% of p53 molecules and 8.0±3.5% of GR molecules as determined directly from the size of these fractions set by our fits ( Table 1 ). Table 1 Parameters obtained from fits to dwell time distributions. Full size table To test if this unique component with the longer dwell times observed within transcription domains required specific-site binding, we performed three control experiments. First, we exploited a distinctive feature of p53 namely that specific- and non-specific-site binding are largely separate functions of the p53 core domain and p53 C-terminal tail, respectively [19] . To disrupt primarily specific-site binding, we generated a mutant (p53-mSB) in which all seven amino acids in the core domain that directly contact the DNA [20] were converted to alanine. We confirmed by PCR with reverse transcription that p53-mSB does not activate p53 target genes ( Supplementary Fig. 3 ). We then measured the distributions of dwell times for p53-mSB within and outside of transcription domains. In accordance with our hypothesis, this distribution of dwell times within transcription domains did not exhibit an extended tail (brown curves in Fig. 3c ) and instead overlapped with the distribution of dwell times outside of transcription domains ( Supplementary Fig. 6a ). A single-component model was sufficient to fit the data for p53-mSB both within and outside of transcription domains and this model yielded similar mean dwell times as wild type (~0.4 s, Table 1 ). We then analysed a well-characterized tumorigenic mutant (p53-R273H) in the core domain [20] . Similar to wild type, longer dwell times were observed only within transcription domains, but the frequencies of longer dwell times were low (green curves in Fig. 3c , Supplementary Fig. 6b ). Fits to the p53-R273H data showed that the fraction of molecules with longer dwell times was reduced from 5.5±1.5% in the wild type to 2.1±2.4% in p53-R273H ( Table 1 ). These data suggest a partial loss of specific-site binding in p53-R273H, consistent with observations that this mutant can still induce some p53-mediated transcription [21] . Finally, as another test of whether the extended tail seen for both wild-type p53 and GR reflected specific-site binding, we compared GR binding using two different ligands with different affinities for GR and with different transcriptional outputs, namely dexamethasone and corticosterone, with the latter being a weaker transcriptional inducer than dexamethasone [22] , [23] . We observed a shorter tail of GR within transcription domains in the presence of corticosterone compared to dexamethasone ( Fig. 3d ). Fitting the GR corticosterone data yielded a shorter residence time (2.8±1.0 s) compared to the GR dexamethasone data (8.1±2.1 s), but the fraction of molecules with longer dwell times remained the same, as did the dwell times of the fast component within transcription domains and the dwell times of the single component outside of transcription domains. Overall, these data support the hypothesis that the unique component with the longer dwell times observed within transcription domains arises from specific-site binding events. Active genes are known to localize within transcription domains, but the identity of the genes found in a randomly selected transcription domain is not known. To increase the specificity of our assay, we measured GR dwell times within the mouse mammary tumor virus (MMTV) tandem array, which contains ~200 MMTV promoters each with 4–6 GR binding sites [3] . Previous work had shown that the array can be visualized by polymerase II labelling in live cells [18] , and that several discrete polymerase II transcription domains associate with the array as detected by BrUTP incorporation [24] . Using an antibody against the polymerase, we confirmed association of the MMTV array with polymerase II foci ( Fig. 4a–c ), and then we performed SMT of GR in the presence of dexamethasone within the transcription domains defined by the association of GFP-polymerase II with the MMTV array ( Fig. 4d ). We observed that the fraction of GR molecules with longer dwell times was substantially larger at the array compared to randomly selected transcription domains ( Fig. 4e ). Fits to the data confirmed these observations, yielding a mean slow fraction of 39±11% within the array compared to 8.0±3.5% within random transcription domains, consistent with the high concentration of specific sites expected at the array ( Table 1 ). 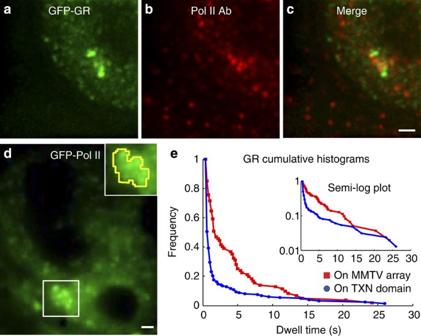Figure 4: GR binding at the MMTV tandem array. The MMTV tandem array (bright green puncta ina) is typically associated with a distinct cluster of polymerase II puncta (b,c). This cluster of polymerase II at the array can also be discerned in live cells (white box ind), and used to define a transcriptionally active zone at the array (yellow outline in the inset). (e) A much higher fraction of molecules with longer dwell times are found at the array compared to randomly selected transcription sites. Scale bar 1 μm. Figure 4: GR binding at the MMTV tandem array. The MMTV tandem array (bright green puncta in a ) is typically associated with a distinct cluster of polymerase II puncta ( b , c ). This cluster of polymerase II at the array can also be discerned in live cells (white box in d ), and used to define a transcriptionally active zone at the array (yellow outline in the inset). ( e ) A much higher fraction of molecules with longer dwell times are found at the array compared to randomly selected transcription sites. Scale bar 1 μm. Full size image We have quantified the residence time and the fraction of transcriptionally productive specific binding of two TFs, GR and p53, at endogenous REs, where transcriptional regulation is known to occur. We used SMT of the TFs within transcriptionally productive domains visualized by GFP-tagged polymerase II. We found that transcriptionally productive binding of both p53 and GR was relatively transient at endogenous REs (3.5±1.6 s for p53 and 8.1±2.1 s for GR), and that only a small fraction of TFs (5.5±1.5% of p53 and 8.0±3.5% of GR) were engaged in transcriptionally productive binding at endogenous REs. The evidence that we detected binding at endogenous REs comes from a comparison of SMT within and outside of transcription domains. We found that within transcription domains a fraction of both p53 and GR molecules exhibited a range of longer dwell times (from ~5 to 25 s), which were not present at other sites in the nucleus that were largely devoid of the polymerase. This unique slow component present within transcription domains is therefore very likely to reflect transcriptionally productive binding at endogenous REs. In support of this, we also observed a disappearance of this component for a stringent specific-site binding mutant of p53, p53-mSB, and a decrease in the size of this component for a moderate specific-site binding mutant of p53, p53-R273H. We also observed a significant increase in the size of this component for GR at the MMTV array where GR-specific binding sites are artificially concentrated, and a significant change in the residence time of GR in the presence of two different ligands with different affinity for the receptor and different transcriptional responses, corticosterone and dexamethasone. This unique component present within transcription domains yielded a mean residence time of 3.5 s for wild-type p53 and 8.1 s for GR in the presence of dexamethasone. This indicates that transcriptionally productive binding of these TFs at endogenous REs occurs with residence times on a time scale of seconds. Note that these residence times may be somewhat underestimated since it is difficult to correct for bleaching of single molecules that remain continuously within the excitation light, but our analysis of histone H2B indicates that photobleaching is not the limiting factor defining our measured residence times for p53 and GR. In addition, the presence of any large tag such as the HaloTag or GFP could also alter residence times. However, our various functional assays such as GR import and p53 gene induction by the tagged molecules show that the tags do not radically alter the functionality of these proteins. Thus, while the true residence times may be somewhat different from our measured residence times, the current measurements are much shorter than the tens of minutes to hour-long residence times originally expected based on in vitro measurements of TF-DNA binding [25] , [26] , and more recently measured in vivo for the TF Rap1 in yeast by a competition ChIP assay [7] . The mean residence times that we measured reflect the average of all residence times of the TF at all the different endogenous REs that are associated with transcription sites. As a result, much complexity is likely to be hidden within this simple average. For example, different REs are likely to have different residence times. Furthermore, it is likely that the binding process at a given RE may involve multiple steps with differing affinities. Dissecting out these various factors will require development of SMT methods that can be repeatedly applied at the same nuclear location to generate large amounts of data, which might then reveal additional binding components or highlight differences in mean residence times at different transcription sites. We found that the residence times of GR at endogenous REs were fairly similar to the residence times at the synthetic MMTV tandem array (8.1±2.1 versus 5.7±0.2 s). The difference between these two estimates could reflect some artificial aspect of the array system, or it could simply reflect that average residence times at the MMTV promoter are in general somewhat shorter than the average residence times over the full range of endogenous GR REs. Overall, this result lends support to the tandem array systems that have been developed as tools for in vivo analysis of transcription. Each of these systems has revealed binding of TFs at specific sites on a time scale of seconds [3] , [4] , [5] , [6] . Together with our current observations, these data continue to raise important questions about how the process of transcription can occur in the face of such transient interactions [1] , [26] . Key issues for future analysis include whether the transient binding event yields a single mRNA transcript or instead marks the endogenous RE for multiple rounds of transcription, and whether other factors required for transcription are simultaneously recruited during the transient binding event or arrive at later times after the TF has departed. Another key question highlighted by our data is how and why different TFs such as GR, p53 and Rap1 can exhibit such large differences in binding residence times at endogenous REs. It is conceivable that some of this disparity could arise from the different techniques applied [2] . The single-molecule approaches are performed in single cells and measure residence times directly from a population of different REs, whereas the competition ChIP approaches are performed on a population of cells and measure residence times indirectly but from the same RE. At the moment, it is uncertain how these technical differences could bias residence time measurements. Thus it seems more likely that residence times may simply range continuously from seconds to tens of minutes depending on the TF and cell type [2] . Consistent with this model are recent measurements using a new technique, cross-linking kinetic (CLK) analysis. While CLK has not yet been applied to site-specific TFs, it has been used to measure intermediate residence times of 1.5–50 min for TATA binding protein at endogenous REs [27] . In addition to the slow binding component found in transcriptionally productive domains with residence times on the order of ~5 s, we also identified a fast component there with a mean dwell time of ~0.3 s for both p53 and GR. We found for both TFs that this same fast component was the sole component present in regions largely devoid of the polymerase. We conclude that the fast component corresponds to processes occurring for both TFs throughout the nucleus. It most likely reflects a combination of slow diffusion events and very transient, presumably non-specific, binding events, processes that are difficult to distinguish experimentally. Given the presence of two components, we also asked what fraction of TF molecules was in the slow component (transcriptionally productive binding at endogenous REs) and what fraction was in the fast component (slow diffusion and non-specific binding). The fits to the dwell time distributions for each TF within transcription domains yielded estimates of 5.5% and 8.0%, respectively, for the fraction of p53 and GR molecules engaged in transcriptionally productive specific-site binding. Since this fraction is absent outside of transcription domains, the percent of total TFs engaged in transcriptionally productive binding can be estimated by multiplying the measured slow fraction for each TF by the fractional nuclear area occupied by the transcription domains in the two cell lines analysed (45±5% in H1299 cells for p53 and 45±5% in 3134 cells for GR). Thus, our data suggest that 0.45 × 5.5%=2.5% of p53 molecules and 0.45 × 8.0%=3.5% of GR molecules are engaged in transcriptionally productive binding. The real percentages might be even smaller, since there could be very weak non-specific binding events or freely diffusing molecules, either of which might disappear faster than we can track with our 10-ms exposure times. On the other hand, the real GR percentages might be higher if the HaloTag version of GR is outcompeted by the endogenous GR. This latter concern does not apply to the p53 estimates, which were obtained in a p53-null cell line, but for p53 we would expect at least some increase in these percentages after stress or DNA damage. Such low fractions of productive TF binding may have important biological consequences. For example, in many cases it could lead to a failure to simultaneously occupy all of the endogenous REs within a single nucleus at any given time [28] . GR has been found by ChIP Seq to have ~10,000 targets in the adenocarcinoma cell line studied here [29] . Thus if only 3.5% of GR molecules are engaged in productive transcription, then to have all 10,000 targets productively occupied in each nucleus ~300,000 GR molecules must be present. This level is at the upper edge of typical TF copy numbers per nucleus, with most TFs expressed at lower numbers [30] , [31] . Such lower copy numbers will yield incomplete occupancy of endogenous REs within the nucleus of each cell. Furthermore, since binding is transient at such REs, the subset of occupied REs will shift with time. This progressive shifting of occupied REs would lead to transcriptional bursting of genes [32] . Response-element occupancy may be a key regulatory feature that could determine whether either a complete or only partial network of genes is operational within an individual cell [2] . Our approach described here can now be used to estimate the fraction of productive binding for other TFs in different cell types and physiological conditions. Constructs and cells We fused the HaloTag to the C-terminus of GR and the N-terminus of p53 under a modified human cytomegalovirus (CMV) intermediate early enhancer/promoter, CMVd1 (Promega). We used a previously described version of a HaloTag H2B in which the N-terminus of H2B is fused with the HaloTag [13] . We transiently co-transfected the GR fusion protein or the H2B fusion protein with GFP-RPB1 (ref. 18) [18] into 3134 cells (which contain the MMTV array [3] ) and the p53 fusion protein with GFP-RPB1 into H1299 cells (which are p53 negative, ATCC CRL-5803) using LipofectamineLTX (Invitrogen) according to the manufacturer’s instructions. We induced GR with 100 nM dexamethasone or 100 nM corticosterone for 25–30 min (except for the experiments on the MMTV array, where we used 100 nM dexamethasone for 45–100 min, which spans the time frame where the arrays in different cells decondense to their maximal extent [33] ). We labelled the fusion proteins with TMR according to our published protocol [13] . Briefly, the cell-permeable fluorescent ligand, HaloTag-TMR ligand (Promega), was added to the wells at concentrations of 5 nM. After an incubation period of 30 min, the cells were washed (3 times for 20 min) with Phenol-red-free complete D-MEM (Invitrogen) to remove the unliganded fluorescent molecules. BrUTP labelling and double labelling of polymerase II and GR at the array have been previously described [24] . Briefly, for BrUTP labelling, the cells expressing GFP-polymerase II were permeabilized in Tris-glycerol buffer (20 mM Tris–HCl, pH 7.4, 5 mM MgCl 2 , 0.5 mM EGTA, 25% glycerol, 25 μg ml −1 digitonin, 1 mM phenylmethylsulphonyl fluoride and recombinant RNasin at 20 U ml −1 ) with 100 nM dexamethasone for 3 min at room temperature. The cells were then incubated for 15 min at room temperature in transcription buffer (100 mM KCl, 50 mM Tris–HCl, pH 7.4, 10 mM MgCl 2 , 0.5 mM EGTA, 25% glycerol, 2 mM ATP, 0.5 mM CTP, 0.5 mM GTP, 0.5 mM BrUTP), 1 mM phenylmethylsulphonyl fluoride and recombinant RNasin at 20 U ml −1 . For double labelling of polymerase II and GR at the array, the cells expressing GFP-GR were fixed in 3.5% paraformaldehyde in PBS for 20 min followed by 0.5% Triton X-100 in PBS for 10 min. After three washes with PBS of 10 min each, the cells were incubated with anti-polymerase II H5 (Covance) overnight at 4 °C. After incubation, washes were performed three times with PBS for a total of 30 min. Then cells were incubated with Cy5-conjugated anti-mouse antibody (Jackson ImmunoResearch Laboratories) for 60 min at room temperature and washed three times in PBS for a total of 20 min. Single-molecule colocalization microscopy We used a custom-built microscope [13] equipped with a 150 × , 1.45 NA objective, a double dichroic, alternating shutter control for 473 and 561-nm lasers and stage with incubator at 37 °C. We used a previously characterized GFP-polymerase II construct to visualize transcription domains [18] . We collected alternate green and red fluorescent images for 20–60 s at the rate of 5 Hz in each channel. Controls with a multicolour fluorescent bead (Tetraspeck, Molecular Probes) demonstrated that there was negligible chromatic aberration in the red and green channels ( Supplementary Fig. 7 ). Data analysis We manually tracked single molecules of GR or p53 in and away from transcription domains. For each experimental condition, we selected 20 regions for tracking from the set of time-lapse movies for that condition. This produced 400–700 tracks per experimental condition, and was sufficient to generate a reasonably smooth cumulative histogram. To increase the odds that the molecules that we measured were actually bound and not diffusing slowly, we only measured dwell times for those molecules that moved <0.3 μm per time point, which is a conservative upper bound for the maximum displacement observed for single molecules of histone H2B bound to chromatin in these cells at this frame rate [13] . We used these measurements to construct dwell time histograms, calculated as the number of molecules with dwell times longer than t . Observational photobleaching was corrected according to our published protocol [13] . Briefly, the photobleaching decay was directly estimated from the single-molecule movies, by plotting the number of detected particles as a function of time. The decay was fit to a bi-exponential decay: , to obtain the photobleaching rates k b,1 and k b,2 together with the corresponding fractions f b,1 and 1− f b,1 . The dwell time histograms were normalized for photobleaching by dividing by B ( t ). Then we fit the dwell time histograms with single- or double-exponential models (see Supplementary Note and Supplementary Fig. 5 ). The equation for single-exponential decay was , where A is a constant, t is time and d 1 is the mean dwell time of the single component. The equation for double-exponential decay was , where f 1 and 1− f 1 are the fraction sizes of the two components with dwell times of d 1 and d 2 . As a test of robustness, the fits were applied to dwell time histograms with progressively more early time points omitted, but this had no significant effect on the basic conclusions (see Supplementary Note and Supplementary Fig. 5 ). To determine the fractional area occupied by transcription sites, for each cell examined we first used ImageJ to draw a region defining the nuclear periphery and then calculated the area of that region that yielded the total nuclear area. Then we used ImageJ to draw regions around each transcription site in that nucleus and then summed the area of all such sites within that nucleus. The latter measurement was divided by the former to yield the fractional nuclear area occupied by transcription sites. Western blotting 3134 cells were transiently co-transfected with Halo-GR and GFP-RPB1 using jetPRIME (Plyplus transfection) according to the manufacturer’s instructions. Note that we changed transfection reagents from the SMT experiments, since virtually all cells were transfected with jetPRIME, enabling a fair comparison of the levels of transfected versus endogenous proteins. By examining the fluorescence signal of GFP-RPB1, we confirmed that expression levels within individual transfected cells were similar between jetPRIME and Lipofectamine LTX. Transfected cells were lysed in RIPA buffer with cOmplete Protease Inhibitor (Roche) and the protein concentration was measured using a Bradford assay (Bio-Rad). Ten micrograms of total proteins was loaded on a 3–8% gradient acrylamide Tris-Acetate gel (Invitrogen) and run for 1 h at 100 V. Proteins were then transferred to a PVDF membrane (Invitrogen) and stained overnight at 4 °C with either anti-GR rabbit antibody (1:5,000, sc-1004, Santa Cruz) or anti-beta-actin rabbit antibody (1:5,000, 13E5, Cell Signaling). HRP-goat anti-rabbit IgG (1:5,000, Invitrogen) was used as a second antibody. The protein of interest was detected using ECL Prime (GE Healthcare). qPCR for mRNA expression Total RNA was prepared from H1299 cells expressing HaloTag only, HaloTag-fused p53 or HaloTag-fused mutant (p53-mSB) with RNeasy (Qiagen) according to the manufacturer’s instructions. Isolated total RNA was then reverse transcribed to cDNA with iScript cDNA Synthesis Kit (Bio-Rad). We performed quantitative PCR on a StepOnePlus (Applied Biosystems) using SYBR green chemistry with the following primer sets, which were described previously [14] : p21 mRNA: forward: 5′-CTGGAGACTCTCAGGGTCGAAA-3′ reverse: 5′-GATTAGGGCTTCCTCTTGGAGAA-3′ MDM2 mRNA: forward: 5′-GTGAATCTACAGGGACGCCATC-3′ reverse: 5′-CTGATCCAACCAATCACCTGAA-3′ PIG3 mRNA: forward: 5′-TCTCTGAAGCAACGCTGAAATTC-3′ reverse: 5′-ACGTTCTTCTCCCAGTAGGATCC-3′. How to cite this article: Morisaki, T. et al. Single-molecule analysis of transcription factor binding at transcription sites in live cells. Nat. Commun. 5:4456 doi: 10.1038/ncomms5456 (2014).